IL-23 promotes TCR-mediated negative selection of thymocytes through the upregulation of IL-23 receptor and RORγt Transient thymic involution is frequently found during inflammation, yet the mode of action of inflammatory cytokines is not well defined. Here we report that interleukin-23 (IL-23) production by the thymic dendritic cells (DCs) promotes apoptosis of the CD4 hi CD8 hi double-positive (DP) thymocytes. A deficiency in IL-23 signalling interferes with negative selection in the male D b /H-Y T-cell receptor (TCR) transgenic mice. IL-23 plus TCR signalling results in significant upregulation of IL-23 receptor (IL-23R) expressed predominantly on CD4 hi CD8 hi CD3 + αβTCR + DP thymocytes, and leads to RORγt-dependent apoptosis. These results extend the action of IL-23 beyond its peripheral effects to a unique role in TCR-mediated negative selection including elimination of natural T regulatory cells in the thymus. The thymic environment orchestrates the development of the diverse repertoire of functional T cells that is required for a robust adaptive immune response to foreign antigens (Ags) while minimizing the generation of T lymphocytes that can attack normal tissues and drive autoimmunity [1] . One key control point in the thymus to maintain self-tolerance involves deletion of those late-stage CD4 + CD8 + double-positive (DP) thymocytes that express autoreactive αβ TCRs and can interact with moderate to high affinity with thymic dendritic cells (DCs) presenting self-Ags [2] , [3] , [4] . Although other antigen-presenting cells in the thymus are involved in negative selection, the high levels of expression of major histocompatibility (MHC) and co-stimulatory molecules on the DCs make them essential for efficient negative selection [5] , [6] , [7] . The synchronized transitions of the gene expression profiles of the developing thymocytes are associated with alterations in the activity of critical transcription factors. One of these, the thymus-specific isoform of the retinoic acid receptor-related orphan receptor (RORγt) is normally only expressed at high levels in early-stage DN and DP thymocytes [8] . It promotes the development and survival of the early-stage DP thymocytes, following expression of the αβTCR, by activating transcription of the gene encoding the anti-apoptotic protein Bcl-xL [9] , [10] , which then inhibits the transcription of c-Rel and Il2 (refs 8 , 11 ). During the later stages of thymocyte development, downregulation of RORγt is essential for the maturation of DP thymocytes into SP thymocytes because RORγt transgene expression in mature T cells affects their multiple functions including enhanced apoptosis and reduced proliferation [8] , [12] , [13] . It has been reported that ectopic overexpression of RORγt results in apoptosis instead of survival of DP in transition to SP thymocytes [14] . Thus, regulation of RORγt can be one factor deciding the fate of late-stage DP thymocytes. The signalling mechanisms that regulate RORγt expression in late-stage DP thymocytes have not been identified. It has been shown that interleukin-23 (IL-23), a highly conserved member of the IL-12 family of regulatory cytokines that is primarily produced by DCs and macrophages [15] , [16] , signals through RORγt in activated CD4 T cells in the periphery [17] , [18] , [19] . In the present study, we investigated whether IL-23 acts through the regulation of RORγt to regulate thymocyte selection. We have made an interesting observation that deficiency of the p19 subunit of IL-23 ( p19 −/− ) significantly reduced thymocyte apoptosis following Aspergillus fumigatus infection in B6 mice. It also perturbed thymic negative selection in male Il23 p19 −/− D b /H-Y T-cell receptor (TCR) transgenic (Tg) mice without affecting thymocyte-positive selection in female Il23 p19 −/− D b /H-Y TCR Tg mice. Overexpression of IL-23 leads to enhanced apoptosis and depletion of late-stage DP thymocytes by upregulation of RORγt and IL-23 receptor (IL-23R) via a TCR/CD3-dependent mechanism. The finding of IL-23-dependent negative selection may indicate a novel central regulation mechanism mediated by a cytokine that is proinflammatory in the periphery. IL-23 drives thymocyte apoptosis during infection IL-23 is important in regulating clearance of pathogens [20] , [21] , [22] , but also is associated with inflammation in autoimmune diseases, multiple sclerosis [23] , [24] , rheumatoid arthritis [25] and lupus [26] . In an attempt to study the anti-fungal effect of IL-23 in clearance of A. fumigatus , we have made a surprising observation that despite the essential role of IL-23 in maintaining host resistance to this pathogen ( Supplementary Fig. 1a ), there was a substantial reduction in thymic size and total thymocyte count on day 4 in normal B6 mice ( Supplementary Fig. 1b ). Terminal deoxynucleotidyl transferase dUTP nick-end labelling (TUNEL) and 7-amino actinomycin D staining indicated that the loss of thymocytes in wild-type (WT) B6 mice was associated with a dramatically increased apoptosis of CD4 + CD8 + DP thymocytes ( Supplementary Fig. 1c,d ). Fluorescence-activated cell sorting (FACS) analysis showed a significant elimination of the CD4 + CD8 + DP population ( Supplementary Fig. 1e ). In contrast, although a deficiency of IL-23 in B6- Il23 p19 −/− mice enhanced A. fumigatus -induced mortality, the massive loss of thymic cellularity and DP thymocytes were largely circumvented ( Supplementary Fig. 1a–e ). Interestingly, IL-23R, which was detected in a small percent of DP thymocytes of naïve mice, was significantly upregulated on day 3 in DP thymocytes of A. fumigatus -infected WT but not B6- Il23 p19 −/− mice ( Supplementary Fig. 1f ). During the course of infection, IL-23 levels were dramatically elevated between days 1–2 ( Supplementary Fig. 1g ). These above findings suggest an interesting concept that IL-23 may potentially affect thymic output. Decreased thymic negative selection in Il23 p19 −/− mice To determine if IL-23 play a role in thymic selection, we crossed Il23 p19 −/− to D b /H-Y TCR Tg background and examined thymocyte negative or positive selection in the male versus female mice, respectively [27] , [28] , [29] , to determine if IL-23 directly plays a role in regulating thymocyte development. In the male mice, the cortical area of the thymus of the Il23 p19 −/− D b /H-Y TCR mice was enlarged compared with the Il23 p19 +/+ D b /H-Y TCR mice ( Fig. 1a ). The thymi were not overtly different in the female Il23 p19 −/− D b /H-Y TCR Tg mice compared with the female Il23 p19 +/+ D b /H-Y TCR Tg mice ( Fig. 1b ). 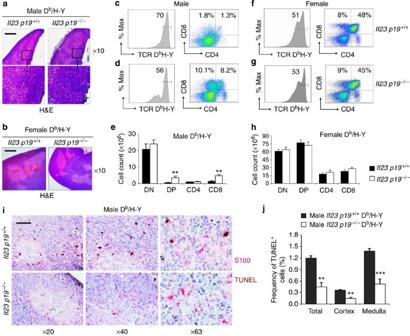Figure 1: Decreased thymic negative selection inIl23 p19−/−mice. (a) Hematoxylin and eosin (H&E) staining of thymus from the indicated male mice. Enlarged images of the outlined area from upper images are shown below. (b) H&E staining of thymus from the indicated female mice. The object lens used to acquire the images is shown. Scale bars inaandb, 300 μm. (c–h) Flow cytometry analysis of the frequency of H-Y TCR+thymocytes and the distribution of CD4/CD8 in H-Y TCR+thymocytes in (c) maleIl23 p19+/+Tg, (d) maleIl23 p19−/−Tg, (f) femaleIl23 p19+/+Tg and (g) femaleIl23 p19−/−Tg mice. In each group, all samples were gated first on Thy1.2+cells. Numbers shown within each quadrant indicate the percent cells in the quadrant. Cell counts of the indicated populations of thymocytes (e,h). All populations were gated within the TCR Db/H-Y+thymocytes. All results shown were calculated based on the percentage of each subpopulation of thymocytes multiplied by the total thymocyte count multiplied by 10−6. (i) Immunohistochemistry staining of thymic DCs (S100+, magenta) and apoptotic cells (TUNEL+, dark brown). The object lens used to acquire each panel of image is shown at the bottom. Scale bar, 100 μm. (j) The percentage of TUNEL+cells at the indicated thymic region was quantified in five randomly chosen microscopic areas from each section. All results represent the mean±s.e.m. (N=2–3 mice per group for three independent experiments; **P<0.01 and ***P<0.005 betweenp19 Il23+/+Db/H-Y Tg male andp19 Il23−/−Db/H-Y Tg male mice). Figure 1: Decreased thymic negative selection in Il23 p19 −/− mice. ( a ) Hematoxylin and eosin (H&E) staining of thymus from the indicated male mice. Enlarged images of the outlined area from upper images are shown below. ( b ) H&E staining of thymus from the indicated female mice. The object lens used to acquire the images is shown. Scale bars in a and b , 300 μm. ( c – h ) Flow cytometry analysis of the frequency of H-Y TCR + thymocytes and the distribution of CD4/CD8 in H-Y TCR + thymocytes in ( c ) male Il23 p19 +/+ Tg, ( d ) male Il23 p19 −/− Tg, ( f ) female Il23 p19 +/+ Tg and ( g ) female Il23 p19 −/− Tg mice. In each group, all samples were gated first on Thy1.2 + cells. Numbers shown within each quadrant indicate the percent cells in the quadrant. Cell counts of the indicated populations of thymocytes ( e , h ). All populations were gated within the TCR D b /H-Y + thymocytes. All results shown were calculated based on the percentage of each subpopulation of thymocytes multiplied by the total thymocyte count multiplied by 10 −6 . ( i ) Immunohistochemistry staining of thymic DCs (S100 + , magenta) and apoptotic cells (TUNEL + , dark brown). The object lens used to acquire each panel of image is shown at the bottom. Scale bar, 100 μm. ( j ) The percentage of TUNEL + cells at the indicated thymic region was quantified in five randomly chosen microscopic areas from each section. All results represent the mean±s.e.m. ( N =2–3 mice per group for three independent experiments; ** P <0.01 and *** P <0.005 between p19 Il23 +/+ D b /H-Y Tg male and p19 Il23 −/− D b /H-Y Tg male mice). Full size image There were a higher percentage and increased cell counts of both DP and CD8 + SP thymocytes in the Il23 p19 −/− D b /H-Y TCR Tg male mice as compared with the Il23 p19 +/+ D b /H-Y TCR Tg male mice, which is consistent with a defect in thymic negative selection ( Fig. 1c–e ). The lack of significant differences in the sizes of the thymocyte subpopulations in the female Il23 p19 +/+ D b /H-Y TCR Tg mice and female Il23 p19 −/− D b /H-Y TCR Tg mice further suggests that IL-23 is not involved in thymic positive selection ( Fig. 1f–h ). The thymic negative selection is a highly specialized process for DP thymocytes that takes place in the thymic medullary areas where tissue-restricted Ags in the periphery are presented. Consistently, the majority of TUNEL + cells were detected in the inner cortex and the medullary area near the vicinity of the thymic S100 + DCs in Il23 p19 +/+ D b /H-Y TCR Tg thymus ( Fig. 1i ). The numbers of the apoptotic cells were dramatically lower in the Il23 p19 −/− D b /H-Y TCR Tg male mice ( Fig. 1i ) and the frequency of apoptotic thymocytes was significantly lower, especially in thymic medullary areas of the Il23 p19 −/− D b /H-Y TCR Tg male than in the Il23 p19 +/+ D b /H-Y Tg male mice ( Fig. 1j ). There was a significantly higher expression of IL-23R on DP thymocytes in Il23 p19 +/+ D b /H-Y TCR Tg male mice comparing with Il23 p19 −/− D b /H-Y TCR Tg male mice ( Supplementary Fig. 2a ). Interestingly, the IL-23R expression on DN thymocytes from both strains are not detectable even those cells have early expression of Tg TCR ( Supplementary Fig. 2a ). Together, these results suggested that there is tight temporal and spatial regulation of IL-23-mediated thymic selection. Decreased thymocyte apoptosis in naïve B6- Il23 p19 −/− mice To further verify our findings, we determined the tissue related expression of Il23 p19 and Il23r in naïve C57BL/6 mice. The results showed that, compared with spleen, lymph nodes, kidney, liver and colon, thymus expresses higher levels of both Il23 and Il23r ( Supplementary Fig. 2b ). Within the different populations of cells sorted from the thymus of naïve B6 mice using the protocol shown in Supplementary Fig. 3 (refs 30 , 31 ), thymic DCs expressed dramatically higher levels of Il23 , compared with cortical epithelial cells and medullary thymic epithelial cells ( Fig. 2a ). Furthermore, Il23r , but not Il23 , mRNA was detectable in Thy1.2 + thymocytes ( Fig. 2b ). Within subpopulations of thymocytes, the levels of Il23r were the highest in CD4 hi CD8 hi DP thymocytes and were almost undetectable in DN and CD8 SP cells ( Fig. 2b ). Il23r was also detected in thymic epithelial cells and DCs ( Fig. 2b ). 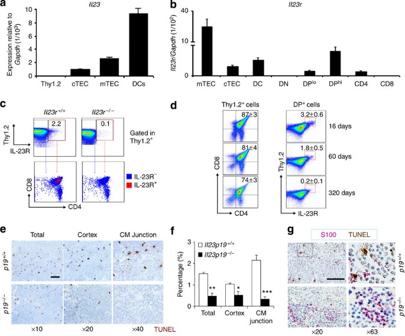Figure 2: Decreased apoptosis in thymus ofIl23 p19−/−mice. (a,b) Quantitative real-time PCR analysis ofIl23(a) andIl23r(b) in the indicated thymic subpopulations of 2-month-old B6 mice. Data are representative of two independent experiments (mean±s.e.m.,N=2–3 mice per experiment). (c) Flow cytometry analysis of IL-23R+thymocyte subpopulation distribution. Thymocytes were gated on Thy1.2+IL-23R+or Thy1.2+IL-23R−separately, each population was analysed for expression of CD4 and CD8. (d) Flow cytometry analysis of IL-23R expression in CD4+CD8+DP thymocyte from mice of the indicated ages. Thymocytes were gated on Thy1.2+population and were analysed for expression of CD4 and CD8 (left). Cells within the DP Thy1.2+subpopulation were analysed for expression of IL-23R (right). (e)In situTUNEL staining on thymus sections ofIl23 p19+/+orIl23 p19−/−C57BL/6J mouse. The magnification of the objective lens used for each panel is shown in the bottom. (f) BioQuant image analysis on the percentage of TUNEL+cells. Five microscopic areas were randomly chosen for the quantitation of each section. Data inc–fare representative of three independent experiments (mean±s.e.m.,N=2–3 mice per group; *P<0.05, **P<0.01, ***P<0.005 betweenIl23 p19+/+andIl23 p19−/−mice). (g)In situstaining of thymic DCs and apoptotic thymocytes using S100 (magenta) and TUNEL staining (brown), respectively. The magnification of the objective lens used for each panel is shown below the images. Scale bar, 100 μm, applies to all panels. Figure 2: Decreased apoptosis in thymus of Il23 p19 −/− mice. ( a , b ) Quantitative real-time PCR analysis of Il23 ( a ) and Il23r ( b ) in the indicated thymic subpopulations of 2-month-old B6 mice. Data are representative of two independent experiments (mean±s.e.m., N =2–3 mice per experiment). ( c ) Flow cytometry analysis of IL-23R + thymocyte subpopulation distribution. Thymocytes were gated on Thy1.2 + IL-23R + or Thy1.2 + IL-23R − separately, each population was analysed for expression of CD4 and CD8. ( d ) Flow cytometry analysis of IL-23R expression in CD4 + CD8 + DP thymocyte from mice of the indicated ages. Thymocytes were gated on Thy1.2 + population and were analysed for expression of CD4 and CD8 (left). Cells within the DP Thy1.2 + subpopulation were analysed for expression of IL-23R (right). ( e ) In situ TUNEL staining on thymus sections of Il23 p19 +/+ or Il23 p19 −/− C57BL/6J mouse. The magnification of the objective lens used for each panel is shown in the bottom. ( f ) BioQuant image analysis on the percentage of TUNEL + cells. Five microscopic areas were randomly chosen for the quantitation of each section. Data in c – f are representative of three independent experiments (mean±s.e.m., N =2–3 mice per group; * P <0.05, ** P <0.01, *** P <0.005 between Il23 p19 +/+ and Il23 p19 −/− mice). ( g ) In situ staining of thymic DCs and apoptotic thymocytes using S100 (magenta) and TUNEL staining (brown), respectively. The magnification of the objective lens used for each panel is shown below the images. Scale bar, 100 μm, applies to all panels. Full size image The specificity of a polyclonal anti-IL-23R antibody was confirmed by analysis on in vitro polarized Th17 and Th1 cells generated from heterozygous IL-23R-green fluorescent protein (GFP) knock-in mouse spleen [32] , [33] ( Supplementary Fig. 4 ). Using this anti-IL-23R antibody, we have identified that IL-23R was expressed by a small percent of thymocytes and the majority of these cells were within the CD4 + CD8 + DP thymocyte population ( Fig. 2c ). The IL-23R + population was almost undetectable in IL-23R-deficient mice ( Fig. 2c ). Interestingly, the percent of this small population of IL-23R + CD4 hi CD8 hi DP thymocytes gradually decreases with increasing age, suggesting the close association with the rate of thymopoiesis ( Fig. 2d and Supplementary Fig. 5 ). We next determined if a deficiency of Il23 was associated with decreased apoptosis. In situ TUNEL staining revealed that the numbers of thymocytes undergoing apoptosis were reduced in Il23 p19 −/− mice compared with WT B6 mice ( Fig. 2e ), and the reduction was apparent especially in the inner cortex and cortical–medullary junction ( Fig. 2f ). The location of TUNEL + thymocytes was determined along with co-staining for S100 + thymic DCs. In WT B6 mice, TUNEL + thymocytes were predominately found in close proximity to the S100 + thymic DCs. In contrast, in Il23 p19 −/− B6 mice, there were fewer TUNEL + apoptotic thymocytes ( Fig. 2g ). These results are consistent with findings derived from A. fumigatus -infected mice or D b /H-Y TCR Tg male mice to suggest that the major function of IL-23R signalling in the thymus is to induce thymocyte apoptosis. Delayed apoptosis induced by IL-23 in the thymus To enable us to follow the kinetics of IL-23-mediated thymocyte apoptosis, exogenous IL-23 was induced by administration of an adenovirus that carries the mouse Il23 gene (AdIL-23) to naïve B6 mice [34] , [35] . An adenovirus carrying the LacZ gene (AdLacZ) was used as a control. The serum levels of IL-23 in the AdIL-23-injected mice were increased over baseline by day 3, reached the maximal value at day 5, were maintained until day 9 and returned to baseline by day 10 ( Supplementary Fig. 6a ). The size of the thymus and its cellularity began to diminish in the AdIL-23-injected mice on day 7 (2 days after the peak level of IL-23 in the sera) ( Fig. 3a and Supplementary Fig. 6b ). Consistent with this, the most significant depletion of the DP thymocytes occurred on day 9 ( Supplementary Fig. 6b ). Flow cytometry analysis revealed that the earliest depletion could be observed in the CD4 hi CD8 hi population 5 days after administration of the AdIL-23 whereas the CD4 lo CD8 lo population became involved somewhat later (by day 7), with the greatest decrease seen at day 9 ( Fig. 3b and Supplementary Table 1 ). Histological staining confirmed a delayed loss of the thymic cortex after AdIL-23 administration ( Fig. 3c and Supplementary Table 2 ). This loss correlated with a dramatically higher level of apoptosis and lower proliferation of thymocytes ( Fig. 3d,e , and Supplementary Table 2 ). z-VAD, a pan-caspase inhibitor, in vivo treatment significantly blocked the IL-23-mediated thymic cellularity loss, which suggests that IL-23 primarily acts through induction of apoptosis to diminish thymus size and thymocyte count in mice ( Supplementary Fig. 7 ). Interestingly, the delayed peak of apoptosis after AdIL-23 does not correlate with the early phase of cytokine induction, and is not observed in control AdLacZ-administered mice. 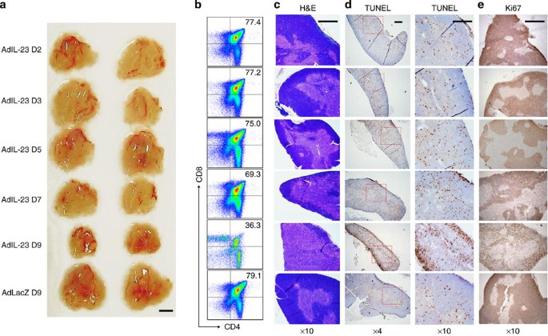Figure 3: Delayed apoptosis induced by IL-23 in the thymus. C57BL/6 mice were injected with either AdIL-23 or AdLacZ. At the indicated day (D), mice were killed. (a) Gross anatomical images of representative thymi from each group of mice. Scale bars, 3.0 mm. (b) Flow cytometry analysis of CD4 and CD8 expression on Thy1.2+cells and the percent of CD4+CD8+cells is shown. (c)In situhematoxylin and eosin (H&E) staining of a representative thymus section. (d)In situTUNEL staining (dark brown) of a representative thymus section. (e)In situKi67 staining (dark brown) of a representative thymus section. The magnification of objective lens used is shown below the images.N=4–5 mice per group for three independent experiments. Scale barsc–e, 300 μm. Figure 3: Delayed apoptosis induced by IL-23 in the thymus. C57BL/6 mice were injected with either AdIL-23 or AdLacZ. At the indicated day (D), mice were killed. ( a ) Gross anatomical images of representative thymi from each group of mice. Scale bars, 3.0 mm. ( b ) Flow cytometry analysis of CD4 and CD8 expression on Thy1.2 + cells and the percent of CD4 + CD8 + cells is shown. ( c ) In situ hematoxylin and eosin (H&E) staining of a representative thymus section. ( d ) In situ TUNEL staining (dark brown) of a representative thymus section. ( e ) In situ Ki67 staining (dark brown) of a representative thymus section. The magnification of objective lens used is shown below the images. N =4–5 mice per group for three independent experiments. Scale bars c – e , 300 μm. Full size image IL-23R is required for IL-23-induced thymocyte apoptosis Based on the finding in A. fumigatus -infected mice that IL-23R upregulation was associated with the massive thymocyte apoptosis, we determined if the delayed onset of exogenous AdIL-23-induced thymocyte apoptosis is related to the requirement of IL-23R upregulation. AdIL-23 or AdLacZ was administered to mice that lack the IL-23R (homozygous IL-23R-GFP knock-in mice) [36] . Neither the reduction in thymus size nor the depletion of DP thymocytes that was observed in AdIL-23-treated WT Il23r +/+ mice was apparent in the AdIL-23-treated Il23r −/− mice ( Fig. 4a,b ; Supplementary Table 3 ). 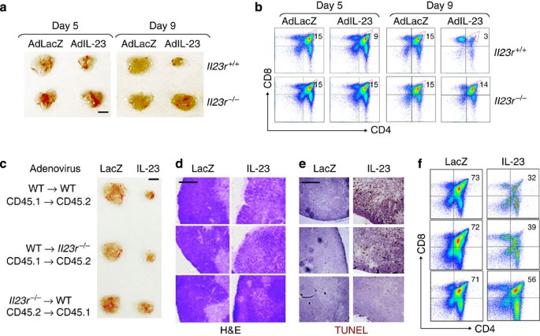Figure 4: Induction of IL-23R for IL-23-induced thymocyte apoptosis. (a,b)Il23r+/+andIl23r−/−mice were administered with either AdIL-23 or AdLacZ. At the indicated time, mice were killed. (a) Gross anatomical images of representative thymi from each group of mice. (b) Flow cytometry analysis of CD4 and CD8 expression on Thy1.2+cells and the percent of CD4+CD8+cells are shown. (c–f) BM reconstitution was carried out in the indicated three groups of donor/recipient chimeric mice. Recipient mice were administered with either AdIL-23 or AdLacZ 40 days later. Mice were killed after 9 days. (c) Gross anatomical images of representative thymi. (d)In situhematoxylin and eosin (H&E) staining of a representative thymus section. (e)In situTUNEL staining (dark brown) of a representative thymus section. (f) Flow cytometry analysis of CD4 and CD8 expression on Thy1.2+cells and the percent of CD4+CD8+cells are shown.N=3 mice per group for two independent experiments. Scale bars ina,c, 3.0 mm; scale bars ind,e, 300 μm. Figure 4: Induction of IL-23R for IL-23-induced thymocyte apoptosis. ( a , b ) Il23r +/+ and Il23r −/− mice were administered with either AdIL-23 or AdLacZ. At the indicated time, mice were killed. ( a ) Gross anatomical images of representative thymi from each group of mice. ( b ) Flow cytometry analysis of CD4 and CD8 expression on Thy1.2 + cells and the percent of CD4 + CD8 + cells are shown. ( c – f ) BM reconstitution was carried out in the indicated three groups of donor/recipient chimeric mice. Recipient mice were administered with either AdIL-23 or AdLacZ 40 days later. Mice were killed after 9 days. ( c ) Gross anatomical images of representative thymi. ( d ) In situ hematoxylin and eosin (H&E) staining of a representative thymus section. ( e ) In situ TUNEL staining (dark brown) of a representative thymus section. ( f ) Flow cytometry analysis of CD4 and CD8 expression on Thy1.2 + cells and the percent of CD4 + CD8 + cells are shown. N =3 mice per group for two independent experiments. Scale bars in a , c , 3.0 mm; scale bars in d , e , 300 μm. Full size image To confirm that IL-23R expression on thymocytes, but not other thymic cells including TEC or DCs that also expressed IL-23R, was essential for IL-23-induced apoptosis, bone marrow (BM) reconstitution was carried out in three conditions (WT→WT, WT→ Il23r −/− and Il23r −/− →WT). In this experimental condition, DCs and macrophages are more susceptible to radiation-induced apoptosis compared with the epithelial cells (CD45 − ) [37] , [38] and thymocytes do not repopulate normally without TECs [39] . We have identified that in all three groups of chimeric mice, there was nearly complete reconstitution of thymocytes, and almost all were derived from transferred donor BM at Day 40 ( Supplementary Fig. 8a,b ). The thymic CD11b + or CD11c + cells, however, remained as recipient origin ( Supplementary Fig. 8c ), suggesting that recipient DCs and TECs remained unaffected under the present experimental condition. AdIL-23 or control AdLacZ was then administered to these three groups of mice. A specific requirement for IL-23R expression on thymocytes to drive apoptosis induced by AdIL-23 is indicated by the dramatic decrease in the sizes of the thymi in both WT→WT and in WT→ Il23r −/− mice compared with Il23r −/− →WT on day 9 after AdIL-23 administration ( Fig. 4c and Supplementary Fig. 8d,e ). A significant loss of the thymic cortex and a higher level of apoptosis were shown in the thymi of AdIL-23-administered recipients from both WT→WT and WT→ Il23r −/− groups compared with Il23r −/− →WT group by histology staining ( Fig. 4d,e ). Depletion of the DP thymocytes was also seen in the thymi of AdIL-23-administered WT→WT and WT→ Il23r −/− groups but was less apparent in those from the Il23r −/− →WT group ( Fig. 4f ). As only thymocytes derived from Il23r +/+ donor cells exhibited high sensitivity to AdIL-23-mediated thymocyte depletion, these results suggest that IL-23R expressed on thymocytes rather than non-thymocytes plays a key role for IL-23-induced thymocyte apoptosis. Consistent with these results, we have identified that AdIL-23 depleted Il23r +/+ thymocytes but spared Il23r −/− thymocytes in recipient mice that have been reconstituted with a 50: 50 ratio of mixed BM from congenically marked CD45.1 Il23r +/+ +CD45.2 Il23r −/− mice ( Supplementary Fig. 9 ), suggesting the high death rate of IL-23R + thymoyctes when encountering IL-23. IL-23 upregulates IL-23R to amplify IL-23-induced apoptosis In peripheral T cells, the expression of IL-23R is induced by their activation and further enhanced by IL-23 (refs 17 , 18 ). Our data showed that only a minor population of DP thymocytes expressed IL-23R under naïve conditions ( Fig. 2c,d and Supplementary Fig. 1f ). To determine if AdIL-23 administration could upregulate IL-23R expression prior to the induction of apoptosis, we examined IL-23R expression within the thymus in vivo at different time points after administration of either AdIL-23 or AdLacZ. The majority of IL-23R + thymocytes were confined to the CD4 hi CD8 hi DP subset and the frequency of these IL-23R + CD4 hi CD8 hi DP thymocytes was significantly higher in the AdIL-23-treated mice than in the AdLacZ-treated mice, especially on day 5 ( Fig. 5a ). Immunofluorescence confocal microscopy analysis showed a dramatic increase of IL-23R + thymocytes in the cortical medulla junction areas of thymus 5 days after AdIL-23 administration ( Fig. 5b ). Four days later, thymocytes that express IL-23R progressed to apoptosis as indicated by an increased population of IL-23R + TUNEL + thymocytes ( Fig. 5b ). We further utilized the heterozygous IL-23R-GFP KI mouse to determine expression of IL- 23R in vivo by GFP fluorescence. Immunofluorescence confocal microscopy analysis indicated that the GFP + cells colocalized with Thy1.2 + cells in the thymus of the AdIL-23-treated IL-23R-GFP KI mice 5 days after treatment ( Fig. 5c,d , right panels). Few GFP + cells can be detected in the thymi of AdLacZ-treated IL-23R-GFP KI mice ( Fig. 5c,d , left panels). These results suggest that AdIL-23 upregulates IL-23R expression and further results in IL-23-mediated apoptosis, which leads to the final loss of IL-23R + subpopulation of thymocytes. 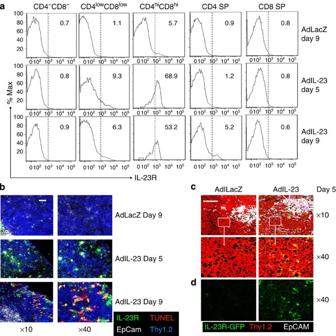Figure 5: IL-23 upregulates IL-23R to further promote IL-23-induced apoptosis. (a) Flow cytometry analysis of IL-23R on the indicated thymocyte populations from WT B6 mice at the indicated times after Ad virus administration. The percent of IL-23R+cells is shown. (b) Immunofluorescent assessment of IL-23R expression by anti-IL-23R (green) and apoptosis (TUNEL, red) of thymic sections from the indicated mice. Sections were co-stained with A647 anti-CD90.2 (blue) and A555 anti-EpCAM (white). Magnification is shown below the images. (c) Immunofluorescent assessment of IL-23R-GFP expression (green) on thymus sections obtained from heterozygousIl23r+/−-GFP KI mice 5 days after either AdLacZ or AdIL-23 administration. Sections were co-stained with anti-CD90.2 (red) and anti-EpCAM (white). Magnification is indicated to the right of the images. (d) A single green channel higher power view of the outlined area fromc.N=4–5 mice per group for three independent experiments. Scale bar, 50 μm, applies to all panels. Figure 5: IL-23 upregulates IL-23R to further promote IL-23-induced apoptosis. ( a ) Flow cytometry analysis of IL-23R on the indicated thymocyte populations from WT B6 mice at the indicated times after Ad virus administration. The percent of IL-23R + cells is shown. ( b ) Immunofluorescent assessment of IL-23R expression by anti-IL-23R (green) and apoptosis (TUNEL, red) of thymic sections from the indicated mice. Sections were co-stained with A647 anti-CD90.2 (blue) and A555 anti-EpCAM (white). Magnification is shown below the images. ( c ) Immunofluorescent assessment of IL-23R-GFP expression (green) on thymus sections obtained from heterozygous Il23r +/− -GFP KI mice 5 days after either AdLacZ or AdIL-23 administration. Sections were co-stained with anti-CD90.2 (red) and anti-EpCAM (white). Magnification is indicated to the right of the images. ( d ) A single green channel higher power view of the outlined area from c . N =4–5 mice per group for three independent experiments. Scale bar, 50 μm, applies to all panels. Full size image IL-23R-RORγt-mediated CD4 hi CD8 hi DP thymocyte apoptosis The roles of RORγt in thymocyte maturation and differentiation have been an interesting question as both RORγt-deficient mice and RORγt transgene (Tg) mice have dramatically decreased cellularity in the thymus [8] , [10] . If IL-23-IL-23R primarily acts on late-stage DP thymocyte apoptosis, this suggests that IL-23 may preferentially regulate the expression of RORγt in late versus early DP thymocytes. Comparison of the transcription levels of Rorc and Il23r in FACS-sorted CD4 hi CD8 hi DP thymocytes and CD4 lo CD8 lo DP thymocytes from either AdLacZ-treated or AdIL-23-treated mice 5 days after treatment revealed that the levels of Rorc and Il23r were similar in FACS-purified CD4 lo CD8 lo DP thymocytes from mice administered with AdIL-23 or AdLacZ ( Fig. 6a ). In contrast, the FACS-purified CD4 hi CD8 hi DP thymocytes from mice administered with AdIL-23 exhibited significantly higher levels of Rorc and Il23r than FACS-purified CD4 hi CD8 hi DP thymocytes from AdLacZ-treated mice ( Fig. 6a ), suggesting that late-stage DP thymocytes are sensitive to AdIL-23-induced upregulation of both Il23r and Rorc. 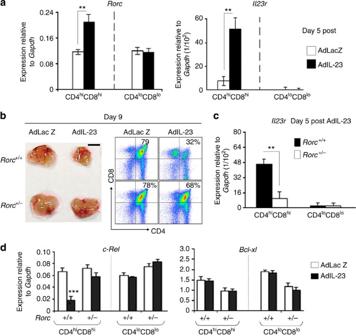Figure 6: CD4hiCD8hiDP thymocytes are targets of IL-23R-RORγt-mediated apoptosis. AdLacZ or AdIL-23 was administered to WT (Rorc+/+) orRorc+/−mice. (a) Quantitative real-time PCR (qRT–PCR) analysis ofRorcandIl23ron the indicated thymocytes ofRorc+/+mice at day 5. (b) Left: Gross anatomic images showing the size of a representative thymus of WT (Rorc+/+) orRorc+/−mice at day 9. Right: Flow cytometry analysis of CD4 and CD8 on total thymocytes (Thy1.2+). The frequency of CD4+CD8+cells within the total Thy1.2+thymocytes is indicated. Scale bar, 3.0 mm. (c) qRT–PCR analysis ofIl23ron the indicated thymocyte subpopulations from the indicated mouse strains at day 5. (d) qRT–PCR analysis of the expression ofc-RelandBcl-xlin the indicated thymocyte subpopulations at day 5. Data in (a–d) are representative of three independent experiments (mean±s.e.m.,N=3–5 mice per group; **P<0.01, ***P<0.005 between AdLacZ and AdIL-23-treated orRorc+/−andRorc+/+mice). Figure 6: CD4 hi CD8 hi DP thymocytes are targets of IL-23R-RORγt-mediated apoptosis. AdLacZ or AdIL-23 was administered to WT ( Rorc +/+ ) or Rorc +/− mice. ( a ) Quantitative real-time PCR (qRT–PCR) analysis of Rorc and Il23r on the indicated thymocytes of Rorc +/+ mice at day 5. ( b ) Left: Gross anatomic images showing the size of a representative thymus of WT ( Rorc +/+ ) or Rorc +/− mice at day 9. Right: Flow cytometry analysis of CD4 and CD8 on total thymocytes (Thy1.2 + ). The frequency of CD4 + CD8 + cells within the total Thy1.2 + thymocytes is indicated. Scale bar, 3.0 mm. ( c ) qRT–PCR analysis of Il23r on the indicated thymocyte subpopulations from the indicated mouse strains at day 5. ( d ) qRT–PCR analysis of the expression of c-Rel and Bcl-xl in the indicated thymocyte subpopulations at day 5. Data in ( a – d ) are representative of three independent experiments (mean±s.e.m., N =3–5 mice per group; ** P <0.01, *** P <0.005 between AdLacZ and AdIL-23-treated or Rorc +/ − and Rorc +/+ mice). Full size image Complete absence of RORγt leads to survival defects of early DP thymocytes [10] and will not be informative to address the selective effects of RORγt in late-stage DP thymocytes. To circumvent this, we utilized heterozygous Rorc +/− mice to determine if lower expression of Rorc could partially rescue CD4 hi CD8 hi thymocytes from AdIL-23-mediated apoptosis ( Fig. 6b ). On day 9 after AdIL-23 or AdLacZ administration, the frequency of DP thymocytes was similar in the control AdLacZ-treated Rorc +/− and Rorc +/+ mice. The frequency of DP thymocytes in the AdIL-23-treated mice Rorc +/− mice was comparable to that in the AdLacZ-treated Rorc +/− mice but was substantially higher than in the AdIL-23-treated Rorc +/+ mice ( Fig. 6b ). The cell count confirmed that DP, especially those CD4 hi CD8 hi thymocytes from Rorc +/− mice are much less sensitive to IL-23-induced apoptosis compared with Rorc +/+ mice ( Supplementary Table 3 ). Moreover, at day 5 post-AdIL-23 treatment, before the dramatic deletion of DP thymocytes, the induction of Il23r in the CD4 hi CD8 hi DP thymocytes from Rorc +/− mice was substantially lower than that in Rorc +/+ mice ( Fig. 6c ). These results suggest that IL-23-mediated induction of RORγt in late-stage CD4 hi CD8 hi DP thymocytes is associated with deletion, but not survival of thymocytes. Target genes of Rorc in the thymus include c-Rel and Bcl-xl (refs 8 , 9 , 10 , 14 , 40 ). Analysis of the CD4 hi CD8 hi DP subset indicated that AdIL-23 treatment was associated with a significant reduction in the levels of c-Rel but did not alter the expression of Bcl-xl in this subset in WT mice ( Fig. 6d ). The levels of both c-Rel and Bcl-xl in the CD4 lo CD8 lo thymocytes were unaffected by AdIL-23 treatment. In contrast, partial deficiency of RORγt prevented AdIL-23-induced suppression of c-Rel in CD4 hi CD8 hi but exhibited no effects of its expression in CD4 lo CD8 lo thymocytes ( Fig. 6d ). Collectively, these results indicate that IL-23 acts through the IL-23R to upregulate RORγt in the late-stage DP thymocytes. Downregulation of the levels of c-Rel is associated with IL-23-induced thymocyte apoptosis in CD4 hi CD8 hi late-stage DP but not CD4 lo CD8 lo early-stage DP thymocytes. Antigen activation initiates the expression of IL-23R Negative selection of thymocytes requires a strong TCR-self Ag interaction [29] . Consistent with the observation that IL-23-mediated thymocytes apoptosis was associated with negative selection, we observed that IL-23R + DP cells expressed higher levels of CD3 and αβTCR as indicated by gating on the IL-23R + population compared with the IL-23R − population ( Fig. 7a ). To determine if loss of TCR stimulation could prevent the upregulation of IL-23R on thymocytes, we administered AdIL-23 to female D b /H-Y TCR Tg mice in which the restricted TCRs were not responsive to all potential endogenous or exogenous Ags during the treatment. Reduction of both the size and cellularity of the thymi were not apparent in female D b /H-Y TCR Tg mice but could be observed in WT female B6 mice 9 days after AdIL-23 treatment ( Fig. 7b ). Histological staining confirmed a significant induction of apoptosis in the thymic cortex of AdIL-23-treated female B6 mice but not D b /H-Y TCR Tg mice ( Fig. 7c,d ). There was no increase of IL-23R + DP thymocytes in the thymi of AdIL-23-treated female D b /H-Y TCR Tg mice compared with thymocytes from the B6 counterparts 9 days after AdIL-23 administration at which time, the CD4 hi CD8 hi population from the thymi of AdIL-23-treated female D b /H-Y TCR Tg mice was almost not affected by IL-23-mediated apoptosis ( Fig. 7e ). 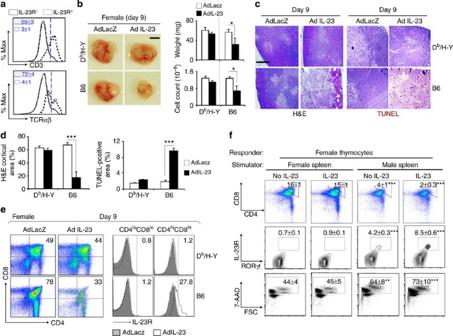Figure 7: Antigen activation initiates the expression of IL-23R on CD4hiCD8hiDP thymocytes. (a) Flow cytometry analysis of the expression of αβTCR and CD3∈on IL-23R+CD4+CD8+or IL-23R−CD4+CD8+thymocytes from naïve C57L/B6J mice. The percentage of αβTCR+or CD3∈cells in the indicated population is shown. (b–e) Female Db/H-Y TCR Tg mice and female C57L/B6J mice were injected with either AdIL-23 or AdLacZ. Mice were killed at day 9. (b) Left: Gross anatomic images showing the size of a representative thymus of the indicated mouse strains. Right: The weight and cellularity are shown. Scale bars, 3.0 mm. (c)In situhematoxylin and eosin (H&E) (left) andin situTUNEL staining (dark brown) (right) of a representative thymus section from the indicated group. The magnification of objective lens is × 10 × . Scale bars, 300 μm. (d) BioQuant quantification of the frequency of thymic cortical area (left) or the frequency of TUNEL-positive area (right) from 10 randomly chosen areas. The results represent mean±s.e.m. (N=2–3 per group for two independent experiments, *P<0.05, **P<0.01, ***P<0.005 for the indicated sample compared with AdLacZ injected group). (e) Left: Flow cytometry analysis of CD4 and CD8 expression on Thy1.2+cells in the indicated group. The percent of CD4+CD8+cells is shown. Right: Flow cytometry analysis of IL-23R on CD4loCD8loand CD4hiCD8hithymocytes. The percentage of IL-23R+cells is indicated. (f) Thymocytes from female Db/H-Y mice were co-culturedin vitrowith irradiated female or male splenocytes from Thy1.1 C57BL/6 in the presence or absence of exogenous mouse recombinant IL-23. Top: Flow cytometry analysis of CD4 and CD8 expression on Thy1.2+cells in the indicated group. The percent of CD4hiCD8hicells is shown; Middle: The expression of IL-23R and RORγt on gated Thy1.2+CD4+CD8+cells is shown; bottom: analysis of apoptosis (7-amino actinomycin D (7-AAD)) in Thy1.2+CD4+CD8+cells. The percent of apoptotic cells is shown (N=3–4 mice per group for two independent experiments; *P<0.05, **P<0.01, ***P<0.005 between thymocytes stimulated with female spleen cells in the absence of IL-23 compared with the indicated group). Figure 7: Antigen activation initiates the expression of IL-23R on CD4 hi CD8 hi DP thymocytes. ( a ) Flow cytometry analysis of the expression of αβTCR and CD3 ∈ on IL-23R + CD4 + CD8 + or IL-23R − CD4 + CD8 + thymocytes from naïve C57L/B6J mice. The percentage of αβTCR + or CD3 ∈ cells in the indicated population is shown. ( b – e ) Female D b /H-Y TCR Tg mice and female C57L/B6J mice were injected with either AdIL-23 or AdLacZ. Mice were killed at day 9. ( b ) Left: Gross anatomic images showing the size of a representative thymus of the indicated mouse strains. Right: The weight and cellularity are shown. Scale bars, 3.0 mm. ( c ) In situ hematoxylin and eosin (H&E) (left) and in situ TUNEL staining (dark brown) (right) of a representative thymus section from the indicated group. The magnification of objective lens is × 10 × . Scale bars, 300 μm. ( d ) BioQuant quantification of the frequency of thymic cortical area (left) or the frequency of TUNEL-positive area (right) from 10 randomly chosen areas. The results represent mean±s.e.m. ( N =2–3 per group for two independent experiments, * P <0.05, ** P <0.01, *** P <0.005 for the indicated sample compared with AdLacZ injected group). ( e ) Left: Flow cytometry analysis of CD4 and CD8 expression on Thy1.2 + cells in the indicated group. The percent of CD4 + CD8 + cells is shown. Right: Flow cytometry analysis of IL-23R on CD4 lo CD8 lo and CD4 hi CD8 hi thymocytes. The percentage of IL-23R + cells is indicated. ( f ) Thymocytes from female D b /H-Y mice were co-cultured in vitro with irradiated female or male splenocytes from Thy1.1 C57BL/6 in the presence or absence of exogenous mouse recombinant IL-23. Top: Flow cytometry analysis of CD4 and CD8 expression on Thy1.2 + cells in the indicated group. The percent of CD4 hi CD8 hi cells is shown; Middle: The expression of IL-23R and RORγt on gated Thy1.2 + CD4 + CD8 + cells is shown; bottom: analysis of apoptosis (7-amino actinomycin D (7-AAD)) in Thy1.2 + CD4 + CD8 + cells. The percent of apoptotic cells is shown ( N =3–4 mice per group for two independent experiments; * P <0.05, ** P <0.01, *** P <0.005 between thymocytes stimulated with female spleen cells in the absence of IL-23 compared with the indicated group). Full size image To further verify that TCR stimulation is necessary for IL-23-induced thymocyte apoptosis machinery, we co-cultured thymocytes from female D b /H-Y TCR Tg mice with irradiated spleen cells from B6 female or male mice in the presence and absence of IL-23. Depletion of CD4 + CD8 + thymocytes and expression levels of RORγt in the thymocytes cultured with irradiated female spleen stimulator cells did not differ with or without IL-23, presumably because the thymocytes lacked IL-23R induced by specific Ag stimulation ( Fig. 7f ). In contrast, co-culture of thymocytes from female D b /H-Y TCR Tg mice with irradiated spleen cells from B6 male mice resulted in a significant upregulation of IL-23R, increased expression of RORγt and increased apoptosis. Furthermore, addition of IL-23 further upregulated both IL-23R and RORγt and greatly enhanced apoptosis ( Fig. 7f ). Similar results were observed after co-culture of MHC class II restricted MOG 35–55 -reactive thymocytes from 2D2 TCR Tg mice with MOG-pulsed irradiated spleen cells in the presence of IL-23 ( Supplementary Fig. 10 ). IL-23 preferentially eliminates natural occurring Treg thymocytes One puzzle is the action of IL-23-mediated deletion of self-reactive T cells in the thymus seem to be in opposition to its well known proinflammatory role in the different autoimmune diseases [23] , [24] , [40] . We thus used Foxp3–GFP mice to track the percent of Foxp3 + Helio + natural occurring Treg (nTreg) cells after AdIL-23 administration. There was a significant reduction of nTregs in CD4 SP cells in the thymus ( Supplementary Fig. 11 ) in the AdIL-23-administered group, comparing with AdLacZ-treated control group. Consistent with these findings, following AdIL-23 administration, in the spleens of WT CD45.1: Il23r −/− CD45.2 mixed BM-reconstituted mice, the nTreg population was primarily Il23r −/− CD45.2 cells, whereas the Th17s were primarily from Il23r +/+ CD45.1 origin ( Supplementary Fig. 12a–f ). These data are consistent with recent studies that high levels of IL-23 was associated with increasing Th17s [40] , [41] , [42] and reduced Tregs [40] , [43] . IL-23 elimination of nTregs in the thymus may therefore act in concert with IL-23 in the periphery to promote autoimmune disease. Our present study advances the present understanding of IL-23 and negative selection in that it implicates IL-23 mediates apoptosis during the process of negative selection in the thymus. The current concept of negative selection is that the induction of apoptosis during negative selection is driven by direct cell contact between the self-antigen-presenting cells and the thymocytes expressing self-reactive TCRs (ref. 44 ). It has been shown that the process of negative selection is less stringent than positive selection because negative selection is never 100% complete and is always associated with some leakage of self-reactive T cells [45] . The present findings are consistent with this variability in that they indicate that while the cell–cell interactions define the specificity of negative selection, IL-23 signalling can act as a second regulatory mechanism that defines the susceptibility of the interacting thymocytes to undergo apoptosis. The current studies do not rule out the possibility that, under some circumstances, higher affinity cell interactions may result in apoptosis in the absence of IL-23 or other cytokine signalling but do suggest that strong IL-23 signalling acts as adjuvant effects to downregulate the threshold of TCR-mediated apoptosis and promotes the elimination of a great proportion of potentially self-reactive thymocytes. The present results suggest that the IL-23-mediated thymocyte apoptosis is under both temporal and spatial regulation. The IL-23 specifically targets the CD4 hi CD8 hi CD3 + αβTCR + late-stage DP thymocyte subset in naïve mice and this highly specific targeting appears to be enforced through several mechanisms. IL-23R expression is limited to a small subset of thymocytes that are phenotypically identical to late-stage DP thymocytes. Within this population, its expression is induced by TCR engagement, suggesting that the interactions with the DCs are a triggering mechanism, and are subsequently enhanced by endogenous IL-23. Moreover, the downstream target of IL-23 signalling of apoptosis is RORγt, a thymus-specific isoform of RORγ, which is expressed predominantly in DP thymocytes [46] . RORγt activates the gene encoding the anti-apoptotic protein Bcl-xL and which has been shown to be required for the survival of early DP thymocytes [10] . Paradoxically, enforced expression of RORγt also lead to dramatic reduction of DP thymocytes [46] . The present findings unify these two apparently contradictory results and directly demonstrate that preferential expression of IL-23R in the late versus early DP thymocytes along with the migration of late DP thymocytes to the IL-23 producing thymic DC area in the medulla lead to differential RORγt-mediated apoptosis versus survival. Furthermore, the IL-23/RORγt-mediated late DP thymocyte apoptosis does not affect the expression of Bcl-xl but is associated with a significant decline in c-Rel . Interestingly, a relatively small change in Rorc was found to exhibit remarkable impact on IL-23R-mediated thymocyte apoptosis. Such results underscore the importance in fine-tuning the expression of Rorc in regulating IL-23 + TCR signalling-induced late-stage DP thymocyte apoptosis. Induction of thymocyte apoptosis by IL-23 overexpression required IL-23R expression, as apoptosis was not increased in treated Il23r −/− mice. Although IL-23R were expressed on different types of cells, the requirement for IL-23R expression on thymocytes but not non-thymocytes for the most efficient IL-23-induced apoptosis was shown by BM reconstitution of CD45.2 Il23r −/− mice with BM from CD45.1 WT mice. Furthermore, in IL-23R-intact mice, 5 days after AdIL-23 administration, IL-23R was highly upregulated on CD4 hi CD8 hi thymocytes, which correlates with the peak levels of IL-23 in the sera and the initial loss of CD4 hi CD8 hi thymocytes. Although IL-23R is predominantly expressed on CD4 hi CD8 hi thymocytes, on subsequent days, there was extensive reduction of both CD4 hi CD8 hi and CD4 lo CD8 lo thymocytes. We proposed that the loss of CD4 hi CD8 hi thymocytes promoted the maturation of CD4 lo CD8 lo thymocytes to CD4 hi CD8 hi thymocytes, which then undergo rapid apoptosis mediated by IL-23. This is supported by the observation that on day 9 after AdIL-23, IL-23R expression colocalized with TUNEL staining, indicating that IL-23R + thymocytes underwent apoptosis. Taken together, we conclude that IL-23 directly induces apoptosis of late-stage DP thymocytes subpopulation. One unexpected finding is the complexity of IL-23R induction and expression on thymocytes. Induction of IL-23R on CD4 hi CD8 hi thymocytes requires antigen stimulation. IL-23R upregulation and the following apoptosis progress were not observed in AdIL-23-treated D b /H-Y TCR Tg female mice due to the lack of H-Y male antigen stimulations. The requirement of TCR engagement for induction of IL-23R was further demonstrated in vitro by co-culture of thymocytes from MHC class I (D b /H-Y, female) or class II (2D2) TCR Tg mice with cells presenting D b /H-Y or H2 b /MOG 35–55 antigen, respectively. However, analysis of IL-23R on DN thymocytes in D b /H-Y TCR Tg male mice shows that despite the early assembling of self-reactive TCR, IL-23R expression is still low, suggesting that assembled TCR complex is required but is not sufficient to induce IL-23-mediated thymocyte apoptosis. A second requirement is signalling through the IL-23R/RORγt pathway that forms a positive feedback loop since IL-23R expression was diminished in Rorc +/− heterozygote mice compared with Rorc +/+ homozygote mice. Thymocyte co-culture in the presence of IL-23 plus self Ag in vitro resulted in further upregulation of IL-23R/RORγt signalling, which lead to IL-23-mediated apoptosis. We therefore propose that under naïve condition, engagement of the TCR complex by self-antigen is a key predisposing factor and IL-23 may act as a second regulatory mechanism to enhance the susceptibility of weakly self-reactive CD4 hi CD8 hi late-stage DP thymocytes to apoptosis. Most thymic cells are able to produce cytokines either spontaneously or after stimulation [47] . Various groups have demonstrated previously that the production of cytokines, such as IL-7 (refs 48 , 49 ) by thymic epithelial cells, IL-12 (ref. 50 ) by thymic DCs as well as IFNγ [51] , [52] , IL-4 (refs 53 , 54 , 55 ) and IL-2 (refs 12 , 56 ) by thymocytes, affects thymocyte development and differentiation. Significant reduction of DP thymocytes was also reported previously under other inflammatory conditions including dextran sulphate sodium-induced colitis [57] , [58] , [59] . We do not completely rule out the involvement of other cytokines in the massive apoptosis found in A. fumigatus -infected mice, although the results suggested that IL-23, in combination with TCR signalling that occurs at the CD4 hi CD8 hi late stage of DP thymocyte development, plays an important role in this process. Increasing evidence suggests that thymic conventional DCs but not plasmacytoid DCs cross-present self-Ags to develop thymocytes and play an important role in thymocyte negative selection and central tolerance induction. All these are consistent with recent finding that CD103 + DCs are the major source of intrathymic IL-23 (ref. 60 ). Our data show for the first time that IL-23 is involved in thymic negative selection. How this process affects multiple cells in the periphery of the host in resolving fungal infection is not precisely known. However, as IL-23R signalling in CD4 + T cells induces effector T H -17 (refs 61 , 62 ) and suppresses regulatory CD4 + T cells [40] in the periphery, our findings suggest a potential IL-23-mediated central immune regulation mechanism that may promote inflammation by limiting thymic regulatory T-cell output. Increased understanding of this process may lead to novel approaches beneficial for control of infection and systemic autoimmune diseases. Mice Il23 p19 −/− mice were obtained from Merck Research Laboratory (Palo Alto, CA) [24] , [25] . The IL-23R-GFP KI mouse and the homozygous Il23r −/− mouse were obtained from the Department of Pediatrics, University of Washington, Seattle, WA [36] . WT B6, B6 C.Cg- Foxp3 tm2Tch /J and B6.129P2(Cg)- Rorc tm2Litt /J [63] mice were obtained from Jackson Laboratory (Bar Harbor, ME) and D b /H-Y Tg from Taconic Farms (Hudson, NY). C57BL/6 CD45.1 (Ly5.1) mice were purchased from the UAB Gnotobiotic Facility. All mice were kept in the animal facilities of University of Alabama at Birmingham, AL, under specific pathogen-free conditions until used for the experiments. All experiments conducted in this study have been reviewed and approved by the institutional animal care and use committee of University of Alabama at Birmingham. All mice were 6–12-week-old female unless otherwise indicated. Preparation of A. fumigatus and in vivo challenge A. fumigatus isolate 13073 was cultured on potato dextrose agar at 37 °C for 7 days, collected with a cell scraper and enumerated using a hemocytometer. 5 × 10 7 A. fumigatus conidia were administrated to each mouse in a volume of 100 μl by intraperitoneal injection. BM transplantation Indicated recipients were sublethally γ-irradiated (320 rads) and reconstituted with indicated donor BM cells. BM cells from donor mice (2 × 10 7 ) were injected into each recipient mouse by intravenous (i.v.) administration 30 min after irradiation. After irradiation, the mice are kept on acidic, antibiotic water for 2 weeks (water is first adjusted to pH 2.6 with concentrated HCl and autoclaved in 1 L bottles. Then, to 1 L of acidic H 2 O, 10 ml of 10 mg ml −1 neomycin in saline (Sigma N112, 20 ml vials) was added. Animals were allowed to recover for at least 5 weeks. Administration of adenovirus and z-VAD For the AdIL-23 producing high expression of IL-23 and the control AdLacZ, AdIL-23 (2 × 10 9 p.f.u. per mouse; a generous gift from Dr Jay K. Kolls at the Louisiana State University Health Sciences Center made by Dr Euan Lockhart) [34] , [35] or AdLacZ (2 × 10 9 p.f.u. per mouse) was administered i.v. z-VAD (200 μg per mouse, R&D, MN) was given by i.v. injection 24 h after AdIL-23 administration. Thymus collection and cell count The thymus was removed and immediately placed in RPMI 1640 medium. Thymi were photographed using a Cool PIX990 digital camera (Nikon, Tokyo, Japan). Single-cell suspensions were obtained after 1% collagenase D (Roche Applied Science, Indianapolis, IN) digestion of whole thymi at 37 °C for 30 min. Thymocyte count was determined using a Cellometer Auto T4 Plus Cell Counter (Nexcelom Biosciences LLC, Lawrence, MA). Flow cytometry analysis Single-cell suspensions of thymocytes were analysed by flow cytometry using combinations of PE-Cy7 anti-mouse CD90.2 (Thy1.2) (1:400 dilution, clone 53-2.1), A700 or APC-anti-CD4 (1:400 dilution, clone H129.19), PE-anti-mouse H-Y TCR (1: 200 dilution, clone T3.70, eBioscience, San Diego, CA), pacific blue anti-mouse CD8 (1:400 dilution, clone 53-6.7), PE-anti-mouse/human Foxp3 (1:50 dilution, clone 150D), APC-anti-mouse/human Helios (1:50 dilution, clone 22F6), Biotin anti-mouse CD3 ∈ antibody (1:400 dilution, clone 145-2C11), Biotin anti-mouse TCR αβ (1:400 dilution, clone WT31, BD Pharmingen, San Diego, CA), Biotin-conjugated anti-CD11c (1:100 dilution, clone N418), APC-anti-human/mouse RORγt (1:100 dilution, clone AFKJS-9, eBioscience) and Anti-IL-23R antibody as primary antibody (1:100 dilution, goat polyclonal to IL23 receptor, Abcam, CA), Alexa Fluor 488 donkey anti-goat IgG (H+L) (1:200 dilution, Invitrogen, CA) as secondary antibody for IL-23R staining. Unless specified, all antibodies used for FACS staining were obtained from BioLegend (San Diego, CA). Single-cell suspensions of thymocytes were washed once with FACS buffer (5% fetal calf serum and 0.1% sodium azide in phosphate-buffered saline (PBS)), and incubated first with unconjugated anti-CD16/CD32 (1:200 dilution, Fc Block; BD Pharmingen) at room temperature for 20 min. Cells were then incubated with a biotin-conjugated Ab at room temperature for 20 min and washed once with FACS buffer. Second-step incubations were performed at room temperature for 20 min with pacific blue, APC-Cy7-streptavidin, PE-, Cy7-, APC- and fluorescein isothiocyanate-conjugated Abs. Intracellular staining for RORγt was performed using the one-step kit for nuclear proteins (eBioscience). After staining, the cells were washed twice with FACS buffer and staining stored in PBS containing 2% paraformaldehyde until FACS analysis. Cells (300,000 per sample) were analysed on an LSRII Flow Cytometry Analyzer (BD Biosciences, Franklin Lakes, NJ). Histology analysis The thymi were removed from the mice immediately after killing, fixed in 10% phosphate-buffered formalin (pH 7.0) and embedded in paraffin. Thin tissue sections (7 nm) were cut, deparaffinated and stained with hematoxylin and eosin. Immunohistochemical staining Tissue samples of the thymi of killed mice were collected and fixed in 10% neutral formalin. Before paraffin sections obtained were stained, endogenous peroxidase activity was suppressed by incubating the slides in 3% H 2 O 2 for 5 min. Sections were incubated in PBS buffer containing 1% BSA, 1 mM EDTA and 0.15 mM NaN3, pH 7.6 with 1% goat serum for 20 min to reduce nonspecific staining. The sections were then incubated for 60 min with the purified rat anti-mouse S100 (1:50 dilution, Clone 6G1, BD Biosciences) diluted in PBE buffer. The secondary reagents were revealed using streptavidin peroxidase (Signet Laboratories, Dedham, MA), which was applied for 20 min. The diaminobenzidine substrate reagent (BioGenex, San Ramon, CA) was prepared immediately before use and applied for 7 min. The stained sections were lightly counterstained with hematoxylin before mounting. In all cases, negative controls, consisting of incubations without the primary Ab, were included in the analyses. TUNEL staining TUNEL staining was performed using an ApopTag In Situ Apoptosis Staining kit on paraffin-embedded sections (Serologicals, Norcross, GA) [63] , [64] . Deparaffinized tissues were quenched in 3.0% hydrogen peroxide for endogenous peroxidase first and then incubate in a humidified chamber at 37 °C for 1 h with Working Strength TdT Enzyme. Anti-digoxigenin conjugate and peroxidase substrate were applied separately for 30 min before mounting. Ki67 staining Thymi were collected and fixed in 10% neutral formalin. Paraffin sections obtained were stained with primary antibodies for Ki67 (1:50 dilution, Laboratory Vision Corporation, Fremont, California). The slides were heated in a 10 mM EDTA solution at pH 8 in a pressure cooker for 10 min and then cooled slowly. Negative controls were performed by omitting the primary antibodies. Secondary detection was accomplished using a multispecies detection system (Signet Laboratories). The sections were exposed to a biotinylated anti-mouse antibody (1:100 dilution) for 20 min and then peroxidase-labelled streptavidin (1:100 dilution) was added for 20 min. A diaminobenzidine tetrachloride supersensitive substrate kit (BioGenex) was used to visualize the antibody–antigen complex. Each section was counterstained using a weak Myer's hematoxylin, dehydrated using graded alcohols and soaked in xylene baths. Frozen fluorescence staining Tissue samples of the thymi of killed mice were embedded in Histo-Prep frozen tissue-embedding medium (Fisher Scientific, Fair Lawn, NJ) and snap-frozen on dry ice. Frozen sections of thymic tissue were fixed in acetone for 15 min before staining. Sections were incubated in PBE buffer (PBS containing 1% BSA, 1 mM EDTA, and 0.15 mM NaN3, pH 7.6) with 1% horse serum for 20 min to reduce nonspecific staining. The sections were then incubated for 30 min with A647 anti-CD90.2 (1:100 dilution, clone 30-H12, BioLegend) and purified anti-EpCAM (clone G8.8, eBioscience) conjugated with A555 by APEX Alex Fluor 555 Antibody Labelling Kit (Invitrogen, CA). In all cases, negative controls, consisting of incubations without the primary Ab, were included in the analyses. Histomorphometry quantitation BioQuant Image Analysis software (R&M Biometrics, Nashville, TN) was used for histomorphometrical analyses as we previously described [24] . On hematoxylin and eosin-stained sections (at × 5), area measurements were made of the total tissue area (area enclosed by the outline of the whole section), cortical area and medullary area (areas distinguished by the difference of the histological appearance and stained colour). Percentages of cortical area and medullary area per total tissue area were calculated using the formula: (cortical area/total tissue area) × 100; and (medullary area/total tissue area) × 100. On TUNEL and Ki67 immunohistochemistry stained sections (at × 5), area measurements were made of the total tissue areas (area enclosed by the outline of the TUNEL-stained section or Ki67-stained section), TUNEL positive and Ki67-positive areas (areas measured by picking the pixels with brown colour from diaminobenzidine chromogen on both sections, using BioQuant’s thresholding tool). Percentages of TUNEL + and Ki67 + area per total tissue area were calculated using the formula: (TUNEL + area/total tissue area) × 100, and (Ki67 + area/total tissue area) × 100. SYBR green real-time quantitative real-time PCR analysis RNA isolated from the thymus of 2-month-old mice (five samples per group) was used to construct cDNA using the Maxima First Strand cDNA Synthesis Kit (Fermentas, Glen Burnie, MD). The sequence of the primers used were: Bcl-xl sense: 5′-GAGCAGGTAGTGAATGAAC-3′, Bcl-xl anti-sense: 5′-GATCCAAGGCTCTAGGTG-3′; Il2 sense: 5′-GAAGGCTATCCATCTCCTCAG-3′, c-Rel anti-sense: 5′-CCTGACACTTCCACAGTTCTTG-3′; Il23 sense: 5′-AGTGTGAAGATGGTTGTGAC-3′, Il23 anti-sense: 5′-CTGGAGGAGTTGGCTGAG-3′; Il23r sense: 5′-CACTGCTGAATGAATGTCCTGGTC-3′; Il23r anti-sense: 5′-GGTATCTATGTAGGTAGGCTTCC-3′; Rorc sense: 5′-TTCTCATCAATGCCAACCG-3′, Rorc anti-sense: 5′-GCCAGTTCCAAATTGTATTGC-3′; Gapdh sense: 5′-AGGTCGGTGTGAACGGATTTG-3′, Gapdh anti-sense: 5′-TGTAGACCATGTAGTTGAGGTCA-3′. All probes were designed to span an intron to prevent amplification of DNA potentially present in the sample. In each run, a series of 10-fold dilutions of a single standard cDNA derived from a positive control mouse RNA (Stratagene, La Jolla, CA) were amplified to create a standard curve, and values of unknown samples were estimated relative to this standard curve. Replicate dilutions of the unknown sample cDNAs from 40 ng of total RNA were combined with a mixture of primers, iQ SYBR Green Supermix with Taq polymerase, and nucleotides (Bio-Rad). Each sample (total volume, 25 μl) was assayed in an optical tube designed for the 96-well format for the IQ5 Thermocycler (Bio-Rad). Each PCR amplification was performed in duplicate using the following conditions: 5 min at 94 °C, followed by a total of 40 cycles (15 s at 94 °C and 30 s at 55 °C). Each PCR was run in duplicate. The mean value of the two reactions was defined as representative of the sample. The volumes described above yielded standard curves with a linear relationship between the copy numbers of the original internal standard added and the number of PCR cycles required to exceed a preset threshold according to the method described by Dreskin et al. [65] From these standard curves, the relative amount of cDNA for the house keeping gene Gapdh and the relative amount of cDNA for each gene were determined for each sample. Thymocyte stimulation assay Thymocytes were cultured in triplicate with IL-2 (5 ng ml −1 , eBioscience) and IL-7 (5 ng ml −1 , R&D), with or without purified mouse rIL-23 (R&D, 20 ng ml −1 ) or irradiated (3,200 rads) splenocytes from male or female Thy1.1 mice as stimulator (ratio: stimulators/responders=1/3) for 20 h. Flow cytometry analysis was performed for the expression of the indicated markers. Apoptosis was quantitated using 7-amino actinomycin D staining and was accessed by flow cytometry [51] . Statistical analysis The values are reported as the mean of each group±s.e.m. Statistical analyses were performed using Student’s unpaired two-tailed t- test. A value of P <0.05 was considered statistically significant. How to cite this article: Li, H. et al. IL-23 promotes TCR-mediated negative selection of thymocytes through the upregulation of IL-23 receptor and RORγt. Nat. Commun. 5:4259 doi: 10.1038/ncomms5259 (2014).